The basis for limited specificity and MHC restriction in a T cell receptor interface αβ T cell receptors (TCRs) recognize peptides presented by major histocompatibility complex (MHC) proteins using multiple complementarity-determining region (CDR) loops. TCRs display an array of poorly understood recognition properties, including specificity, crossreactivity and MHC restriction. Here we report a comprehensive thermodynamic deconstruction of the interaction between the A6 TCR and the Tax peptide presented by the class I MHC HLA-A*0201, uncovering the physical basis for the receptor’s recognition properties. Broadly, our findings are in conflict with widely held generalities regarding TCR recognition, such as the relative contributions of central and peripheral peptide residues and the roles of the hypervariable and germline CDR loops in engaging peptide and MHC. Instead, we find that the recognition properties of the receptor emerge from the need to engage the composite peptide/MHC surface, with the receptor utilizing its CDR loops in a cooperative fashion such that specificity, crossreactivity and MHC restriction are inextricably linked. Recognition of peptide antigens by the αβ T cell receptor (TCR) underlies cellular immunity. TCRs recognize peptides bound and presented by major histocompatibility complex (MHC) proteins, using multiple complementarity-determining region (CDR) loops to contact the composite peptide-MHC surface (pMHC). A notable aspect of the TCR–pMHC interaction is that the distribution of binding energy within the interface has significant functional implications. The immune response is directed towards the peptide, yet TCRs invariably contact both peptide and MHC. It is commonly expected that contacts between the TCR and peptide should be stronger than those between TCR and MHC to ensure antigen specificity. Within this framework, the various CDR loops have often been ascribed ‘roles’ in TCR recognition, with weak recognition of the MHC attributed to the germline-encoded CDR1 and CDR2 loops and recognition of the peptide attributed to the hypervariable CDR3 loops. While this view logically pairs the diverse and genetically conserved regions of the TCR–pMHC interface (peptide with CDR3; MHC with CDR1/CDR2), such simplifying distinctions are rarely evident in TCR–pMHC crystallographic structures [1] . Several studies have attempted to address the energetic contributions of different interfacial regions to TCR–pMHC binding through mutagenesis, and alanine scans of both receptor and ligand have been performed [2] , [3] , [4] , [5] . Varying conclusions from these studies together with the growing number of TCR–pMHC structures have indicated that the energetic contributions of regions will likely vary among TCR–pMHC interfaces [6] . Thus, alanine scans have been followed with more targeted substitutions, aiming to identify trends that might yield insight into phenomena such as MHC restriction, peptide specificity or TCR crossreactivity. However, while single mutagenesis is useful for examining regions that influence binding and specificity, single mutations cannot probe the strengths of pairwise interactions and provide poor estimates of the contributions of sidechains to binding affinity. These caveats have been reviewed in detail [7] , and in one case resulted in incorrect conclusions regarding TCR specificity [8] . More direct measurements of energetic contributions to binding are obtainable from double-mutant cycles, which can account for both structural and energetic responses to mutations and permit the direct probing of the strengths of interactions between sidechains [9] . Here, we utilize double-mutant cycles to dissect the interface between the αβ TCR A6 and its best studied ligand, the Tax peptide presented by the class I MHC HLA-A*0201 (HLA-A2). The significant amount of structural, biophysical and functional data available for the A6 TCR provided context in which to interpret the measurements. For comparison, select measurements are repeated with two additional TCR–pMHC pairs. Our observations, several of which conflict with widely held generalities regarding TCR recognition, shed new light on the origin of TCR-limited specificity and MHC restriction, two defining features of TCR recognition for which a variety and sometimes competing explanations have been offered. Conclusions applicable to TCR recognition in general relate to the role of hypervariable loop flexibility in promoting limited rather than tight specificity, and that TCR specificity and MHC restriction can be inextricably linked, the latter reflecting the fact that the TCR must engage a composite peptide/MHC ligand with tightly coupled structural properties. Double-mutant cycles in the A6 TCR—Tax/HLA-A2 interface We began by identifying all interacting sidechains in the interface between the A6 TCR and Tax/HLA-A2 (ref. 10 ). There are 21 such pairs, involving 16 amino acids of the TCR, 10 of HLA-A2 and 3 of the peptide. The interaction free energy ( ) between each pair was measured via double-mutant cycles. Including controls, 38 cycles in the A6-Tax/HLA-A2 interface were performed. Eight additional cycles were performed in the interfaces between the B7 TCR and Tax/HLA-A2 and the DMF5 TCR and MART-1 26(27L)-35 /HLA-A2. The data were collected and analysed using a strategy in which all four measurements of a cycle were performed in a single surface plasmon resonance experiment and the data fit globally. This approach substantially increased sensitivity and improved accuracy and reproducibility compared with the traditional approach in which cycles are constructed from independently measured values. A representative double-mutant cycle is shown in Fig. 1a , and the results of all cycles are listed in Supplementary Tables S1 and S2 . Errors in the measurements ranged from ±0.1 to ±0.5 kcal mol −1 , with an average error of ±0.1 kcal mol −1 . Reproducibility was excellent: each cycle included two replicates, and seven cycles were performed at least two additional times. In all but one case the values for repeated cycles were identical within error, and in the single outlying case the values were weak. In all but one easily rationalized case, cycles repeated with different amino acids (for example, separate cycles with alanine and phenylalanine substituted for pTyr5) yielded identical conclusions. Control cycles performed between residues whose sidechain atoms were far apart and not poised to interact yielded values of zero within error. The average Δ G ° for the interaction between wild-type A6 and Tax/HLA-A2 was −7.6±0.1 kcal mol −1 , in excellent agreement with values determined previously [11] , [12] . 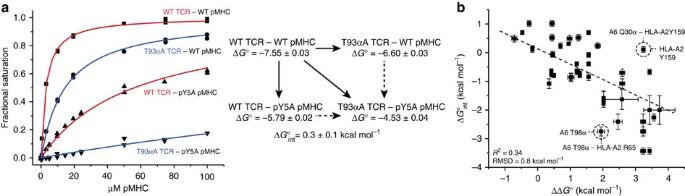Figure 1: Double-mutant cycles in the A6-Tax/HLA-A2 interface. (a) Data for all four interactions defining a double-mutant cycle (in this example, the A6 T98α—Tax/HLA-A2 pY5 interaction) were collected in one experiment, in which duplicate concentration series of wild-type or mutant pMHC were injected over adjacent flow cells coupled with wild-type or mutant TCR. All eight data sets were fit globally to a model in which the surface activities for the four data sets over the wild-type TCR surface (indicated with red) and the four data sets over the mutant TCR surface (indicated with blue) were shared parameters. Construction of the double-mutant cycle and the resulting interaction free energy for the T98α—pY5 interaction are shown to the right of the plot. (b) For cycles in the A6-Tax/HLA-A2 interface, plotting the free energy of interaction of each residue () versus the effect of its mutation on the binding free energy (ΔΔG°) showed that while the most destabilizing mutations were generally involved in the strongest interactions, the results were poorly correlated. Two data points that illustrate the poor correlation are highlighted: the hydrogen bond between Thr98α of A6 and Arg65 of HLA-A2 is stronger than predicted by the ΔΔG° of the T98αA mutation, and the van der Waals interaction between Gln30α of A6 and Tyr159 of HLA-A2 is almost negligible, despite the large ΔΔG° for the Y159A mutation. Error bars reflect standard parameter error from the global fits of eight data sets. Figure 1: Double-mutant cycles in the A6-Tax/HLA-A2 interface. ( a ) Data for all four interactions defining a double-mutant cycle (in this example, the A6 T98α—Tax/HLA-A2 pY5 interaction) were collected in one experiment, in which duplicate concentration series of wild-type or mutant pMHC were injected over adjacent flow cells coupled with wild-type or mutant TCR. All eight data sets were fit globally to a model in which the surface activities for the four data sets over the wild-type TCR surface (indicated with red) and the four data sets over the mutant TCR surface (indicated with blue) were shared parameters. Construction of the double-mutant cycle and the resulting interaction free energy for the T98α—pY5 interaction are shown to the right of the plot. ( b ) For cycles in the A6-Tax/HLA-A2 interface, plotting the free energy of interaction of each residue ( ) versus the effect of its mutation on the binding free energy (ΔΔ G °) showed that while the most destabilizing mutations were generally involved in the strongest interactions, the results were poorly correlated. Two data points that illustrate the poor correlation are highlighted: the hydrogen bond between Thr98α of A6 and Arg65 of HLA-A2 is stronger than predicted by the ΔΔ G ° of the T98αA mutation, and the van der Waals interaction between Gln30α of A6 and Tyr159 of HLA-A2 is almost negligible, despite the large ΔΔ G ° for the Y159A mutation. Error bars reflect standard parameter error from the global fits of eight data sets. Full size image The ΔΔ G ° values resulting from single mutations were poorly correlated with the values involving the same sites ( Fig. 1b ). Generally, the most destabilizing single mutations were involved in the most favourable interactions, but quantitatively the ΔΔ G ° values from the single mutations were poor predictors of the strengths of these interactions. We found several cases where single mutations had significant effects on binding, yet the mutated sites participated in interactions that were either negligible or weakly unfavourable, or vice versa. Two examples are highlighted in Fig. 1b : the hydrogen bond between Thr98α of A6 and Arg65 of HLA-A2 is significantly stronger than predicted by the ΔΔ G ° of the T98αA mutation, and the van der Waals interaction between Gln30α of A6 and Tyr159 of HLA-A2 is almost negligible, despite the large ΔΔ G ° for the Y159A mutation. Interactions at the periphery dominate peptide contributions In the A6-Tax/HLA-A2 structure, eight sidechains of the TCR interact with three of the peptide. The majority of the interactions are made with pTyr5, which lies at the centre of the interface and is accommodated in a pocket formed by the TCR α and β chains ( Fig. 2a ). Two hydrogen bonds are formed to the tyrosine hydroxyl, one between Ser31 of CDR1α and one with Arg95 of CDR3β. Only the hydrogen bond with Ser31α was significant ( of −0.9 kcal mol −1 ). The strength of the hydrogen bond with Arg95β was negligible at −0.2 kcal mol −1 , likely owing to the entropic cost of ordering the flexible CDR3β loop [13] . The remaining interactions with pTyr5 ranged from weakly favourable to unfavourable. Summing the various values leads to a negligible contribution of −0.1 kcal mol −1 for the interactions with the tyrosine sidechain. The data thus indicate that contacts to tyrosine 5 contribute a negligible amount to the affinity of A6 towards Tax/HLA-A2, despite the position of the sidechain in the centre of the interface. Note that summation of the values assumes additivity between the double-mutant cycles, an assumption subjected to caveats as described below. However, the results explain the ability of T cells expressing A6 to recognize targets presenting Tax variants with a wide range of amino acids substituted for pTyr5, including alanine and bulky non-natural amino acids [14] , [15] . 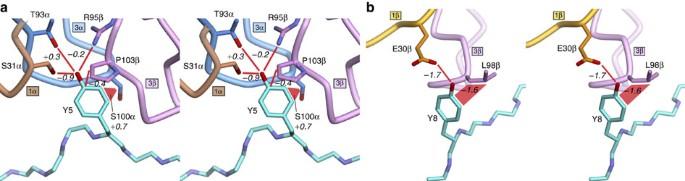Figure 2: Cross-eyed stereo views of the interactions between the position 5 and position 8 tyrosines of the Tax peptide and sidechains of the A6 TCR. (a) Engagement of pTyr5 at the centre of the interface by sidechains of CDR1α, CDR3α and CDR3β contributes little to TCR affinity. Interactions between sidechains are highlighted by red lines, and the free energies of each interaction are indicated in units of kcal mol−1. (b) In contrast with pTyr5, engagement of pTyr8 by sidechains of CDR1β and CDR3β contributes significantly to TCR affinity. Figure 2: Cross-eyed stereo views of the interactions between the position 5 and position 8 tyrosines of the Tax peptide and sidechains of the A6 TCR. ( a ) Engagement of pTyr5 at the centre of the interface by sidechains of CDR1α, CDR3α and CDR3β contributes little to TCR affinity. Interactions between sidechains are highlighted by red lines, and the free energies of each interaction are indicated in units of kcal mol −1 . ( b ) In contrast with pTyr5, engagement of pTyr8 by sidechains of CDR1β and CDR3β contributes significantly to TCR affinity. Full size image The sidechain of pLeu1 forms a single van der Waals interaction with the sidechain of Gln30 of CDR1α. The Q30A variant of the A6 α chain expressed poorly, prohibiting a cycle with alanine at this position. However, substitutions with leucine and valine could be made, both yielding an almost negligible of +0.2 kcal mol −1 . Consistent with this result, A6 T cells are widely tolerant of substitutions to pLeu1 (ref. 14 ). As opposed to pTyr5, pTyr8 is at the periphery of the interface and only interacts with two sidechains of A6. A hydrogen bond is formed between the pTyr8 hydroxyl and the sidechain of Glu30 of CDR1β, and van der Waals contacts are formed between the tyrosine ring and the sidechain of Leu98 of CDR3β. Both interactions were found to be unusually strong ( Fig. 2b ): the for the pTyr8–Glu30β hydrogen bond was measured as −1.7 kcal mol −1 , and the for the interactions with Leu98β was measured as −1.6 kcal mol −1 . The hydrogen bond measurement was repeated twice, first in the background of an affinity-enhancing modification to the pTyr5 sidechain [16] , and second with a phenylalanine substitution at position 8. Both measurements yielded results identical within error to the first. The strength of the hydrogen bond likely arises because both pTyr8 and Glu30β remain solvent-exposed after forming the TCR–pMHC complex, minimizing the desolvation penalty that occurs upon hydrogen bond formation [17] . Overall, the data indicate that the sidechain of pTyr8 dominates the peptide side contribution to TCR-binding affinity. This dominance is reflected in functional measurements with A6 T cells, which tolerate substitutions to the sidechain of tyrosine 8 poorly [14] . Further, unlike interactions to the centre of the peptide, the interactions between the TCR and pTyr8 are conserved across all ten crystal structures of A6 bound to different peptide/HLA-A2 complexes [10] , [12] , [13] , [15] , [16] , [18] , [19] . Interactions with CDR3α dominate α1 helix contributions Five sidechains of the A6 CDR1α and CDR3α loops interact with a range of sidechains across the HLA–A2 α1 helix. The values were dominated by extremely favourable interactions between the sidechains of Thr98 and Asp99 of CDR3α and Arg65 of the HLA-A2 α1 helix ( Fig. 3a ). The strength of the hydrogen bond between Thr98α and Arg65 was measured as −2.8 kcal mol −1 . The salt bridge between Asp99α and Arg65 was even stronger, with two independent measurements of −3.4 and −3.0 kcal mol −1 . These measurements could only be made with the aid of affinity-enhancing substitutions in CDR3β (ref. 20 ). However, a cycle could be performed without using an altered CDR3β by mutating position 99 to an asparagine rather than alanine. In that case, the value was still an exceptionally strong −2.5 kcal mol −1 . Engagement of Arg65 thus contributes a remarkable degree of favourable binding free energy: assuming additivity between the cycles, the total amounts to −5 to −6 kcal mol −1 . The interactions between Arg65 and residues of the hypervariable CDR3α loop account for the largest energetic contributions measured in the A6-Tax/HLA-A2 interface. The substantial contributions may reflect an optimal electrostatic environment together with the reduced desolvation penalty required for burial of an arginine [21] . 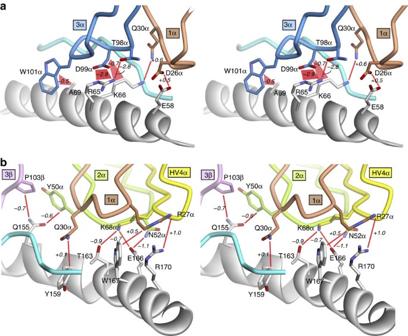Figure 3: Cross-eyed stereo views of the interactions between sidechains of the HLA-A2 α1 and α2 helices and those of the A6 TCR. (a) Recognition of the HLA-A2 α1 helix by sidechains of CDR1α and CDR3α is dominated by interactions between Arg65 and the sidechains of Thr98α and Asp99α of the CDR3α loop. The remainder of the interactions range from moderately unfavourable to moderately favourable. Interactions between sidechains are highlighted by red lines, and the free energies of each interaction are indicated in units of kcal mol−1. (b) Recognition of the HLA-A2 α2 helix by sidechains of CDR1α, CDR2α, CDR3β and HV4α proceeds via a range of moderately favourable to moderately unfavourable interactions. Figure 3: Cross-eyed stereo views of the interactions between sidechains of the HLA-A2 α1 and α2 helices and those of the A6 TCR. ( a ) Recognition of the HLA-A2 α1 helix by sidechains of CDR1α and CDR3α is dominated by interactions between Arg65 and the sidechains of Thr98α and Asp99α of the CDR3α loop. The remainder of the interactions range from moderately unfavourable to moderately favourable. Interactions between sidechains are highlighted by red lines, and the free energies of each interaction are indicated in units of kcal mol −1 . ( b ) Recognition of the HLA-A2 α2 helix by sidechains of CDR1α, CDR2α, CDR3β and HV4α proceeds via a range of moderately favourable to moderately unfavourable interactions. Full size image The remaining interactions between the TCR and the α1 helix of HLA-A2 ranged from moderately favourable to weakly unfavourable. The two interactions between the germline CDR1α loop and the α1 helix were unfavourable, with values of +0.5 kcal mol −1 (Asp26α—Glu58) and +0.6 kcal mol −1 (Gln30α—Lys66). Interactions with the α2 helix are at best moderate Six sidechains of the A6 TCR, including those from CDR1α, CDR2α, HV4α and CDR3β, interact with eight sidechains across the HLA–A2 α2 helix ( Fig. 3b ). Unlike the interactions with the peptide or the α1 helix, the interactions between the TCR and the α2 helix were not dominated by highly favourable interactions, but rather had values distributed between moderately favourable and moderately unfavourable. The interactions between sidechains of CDR1α and the α2 helix were all unfavourable, with values of +0.1, +0.5 and +1.0 kcal mol −1 . These repulsive interactions were balanced by favourable interactions between sidechains of CDR2α and the α2 helix, consisting of hydrogen bonds with strengths of −1.0 and −0.7 kcal mol −1 . The interaction between Tyr50 of CDR2α and Gln155 of the α2 helix is of interest given descriptions of conserved interactions occurring between germline loops of TCRs and the α helices of MHC proteins [22] , [23] . The A6 TCR shares the Vα 12-2 domain with two other TCRs that have been crystallized with peptide/HLA-A2 complexes [24] , [25] . Although there are no conserved contacts between the TCRs and HLA-A2 in these structures, there is a shared pattern of interactions involving Tyr50 of CDR2α and Gln155 (ref. 24 ). The interaction between Tyr50α and Gln155 in the A6-Tax/HLA-A2 was indeed favourable, although only moderately so, with a of −0.6 kcal mol −1 . The adjacent hydrogen bond between Asn52 of CDR2α and Glu166 of the HLA-A2 α2 helix was more favourable at −1.1 kcal mol −1 , but this hydrogen bond is not conserved in the three Vα 12-2 TCR-peptide/HLA-A2 interfaces [24] . The interactions between the HV4α loop and HLA-A2, involving electrostatic interactions between Lys68α and Thr163 and Glu166, were moderate, with interaction free energies of −0.9 and −0.7 kcal mol −1 , respectively. The sole interaction between CDR3β and the α2 helix, between Pro103β and Gln155, was also moderate, with a of −0.7 kcal mol −1 . Contributions tabulated by interface component The values from the double-mutant cycles in the A6-Tax/HLA-A2 interface are arranged according to CDR loop in Fig. 4 . The extremely favourable interactions between sidechains of CDR3α and the HLA-A2 α1 helix are especially clear, as are the favourable interactions between sidechains of the two CDR1 loops and the peptide. Also of interest are the opposing interactions between the peptide and CDR3α (unfavourable), and the peptide and CDR3β (favourable). Note that the summation in Fig. 4 assumes additivity with caveats as discussed below. However, as noted earlier the results explain a wealth of functional data, and the distribution in Fig. 4 agrees well with computational calculations on the distribution of energy in the A6-Tax/HLA-A2 interface [26] . 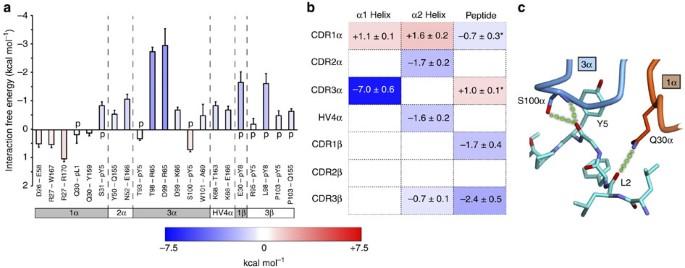Figure 4: Summary of the double-mutant cycle results for the A6 TCR and the contributions of various interfacial regions to binding. (a) Results of each cycle grouped by CDR loop. Cycles involving a peptide sidechain are indicated with a ‘p’ in the graph. Error bars reflect standard parameter error from the global fits of eight data sets. (b) Contributions to the overall binding free energy of the A6 TCR tabulated by interfacial region. As discussed in the text and as indicated within an asterisk, the contributions of CDR1α and CDR3α are likely an underestimate due to the presence of hydrogen bonds from residues of these loops to the backbone of the Tax peptide. In panelsaandb, the interaction free energies are coloured according to the scale at the bottom, with blue reflecting favourable interactions and red unfavourable. Errors in panelbreflect propagated error from values in panelaandSupplementary Tables S1 and S2. (c) Hydrogen bonds involving backbone atoms in the interface between the A6 TCR and Tax/HLA-A2. Figure 4: Summary of the double-mutant cycle results for the A6 TCR and the contributions of various interfacial regions to binding. ( a ) Results of each cycle grouped by CDR loop. Cycles involving a peptide sidechain are indicated with a ‘p’ in the graph. Error bars reflect standard parameter error from the global fits of eight data sets. ( b ) Contributions to the overall binding free energy of the A6 TCR tabulated by interfacial region. As discussed in the text and as indicated within an asterisk, the contributions of CDR1α and CDR3α are likely an underestimate due to the presence of hydrogen bonds from residues of these loops to the backbone of the Tax peptide. In panels a and b , the interaction free energies are coloured according to the scale at the bottom, with blue reflecting favourable interactions and red unfavourable. Errors in panel b reflect propagated error from values in panel a and Supplementary Tables S1 and S2 . ( c ) Hydrogen bonds involving backbone atoms in the interface between the A6 TCR and Tax/HLA-A2. Full size image In addition to global effects, including changes in flexibility that propagate away from the binding sites [27] and the loss in rotational/translational entropy that occurs upon binding (estimated at 4–6 kcal mol −1 ) [28] , [29] , a notable component missing from our analysis is interactions with backbone atoms, which cannot be probed by double-mutant cycles. Within the A6-Tax/HLA-A2 interface there are three backbone-mediated hydrogen bonds, all to the peptide ( Fig. 4c ). Two are between the carbonyl oxygen of pGly4 and Ser100 of CDR3α. The third is between the carbonyl oxygen of pLeu2 and Gln30 of CDR1α. The majority of hydrogen bonds within protein structures have been found to be modestly favourable (a recent analysis of double-mutant cycles found an average strength of −0.5 kcal mol −1 (ref. 30 )). Our analysis thus likely underestimates the favourable contributions of CDR1α and CDR3α to recognition of the Tax peptide, but not to an extent that would alter our conclusions. Shared interactions between Vα 12-2 TCRs and HLA-A2 are weak As noted above, Tyr50 of CDR2α and Gln155 of HLA-A2 share a pattern of interactions in three Vα 12-2 TCR-peptide/HLA-A2 interfaces [29] , [30] . We therefore probed the interaction between Tyr50α and Gln155 in the interface between the Vα 12-2 TCR DMF5 and its MART-1 26(27L)-35 /HLA-A2 ligand. The strength of this interaction was identical to that measured in the A6 interface, with a weak of −0.6 kcal mol −1 ( Fig. 5 ). We also probed the interaction between Asn52α and Glu166 in the DMF5 interface, as these sidechains also interact in both the A6 and DMF5 interfaces, although the hydrogen bond is not present with DMF5. Consistent with the structural differences, the strength of the interaction was weaker in the DMF5 interface, with a of only −0.3 kcal mol −1 with DMF5 (compared with −1.1 kcal mol −1 with A6). 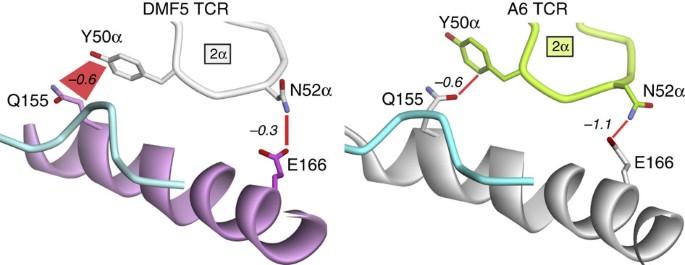Figure 5: Comparison of CDR2α—HLA-A2 interactions conserved in two Vα 12-2 TCR interfaces. In the DMF5 interface, the interaction between Tyr50 of CDR2α and Gln155 is weakly stabilizing, with aof −0.6 kcal mol−1. This is identical to the strength of the Y50α–Q155 interaction in the A6 interface. The interaction between Asn52 of CDR2α and Glu166 is weak in the DMF5 interface, with aof −0.3 kcal mol−1. The interaction is much stronger in the A6 interface, with aof −1.1 kcal mol−1. Figure 5: Comparison of CDR2α—HLA-A2 interactions conserved in two Vα 12-2 TCR interfaces. In the DMF5 interface, the interaction between Tyr50 of CDR2α and Gln155 is weakly stabilizing, with a of −0.6 kcal mol −1 . This is identical to the strength of the Y50α–Q155 interaction in the A6 interface. The interaction between Asn52 of CDR2α and Glu166 is weak in the DMF5 interface, with a of −0.3 kcal mol −1 . The interaction is much stronger in the A6 interface, with a of −1.1 kcal mol −1 . Full size image Analysis of the B7 TCR supports conclusions drawn from A6 The B7 TCR also recognizes the Tax peptide presented by HLA-A2, allowing us to ask to what extent observations made with A6 are shared with B7. As with A6, the B7 TCR accommodates the pTyr5 sidechain in a pocket formed by the CDR3α and CDR3β loops. However, the two pockets have opposing electrostatics: the pocket is positively charged in A6, whereas in B7 it is negatively charged owing to the presence of Asp30 of B7 the CDR1α loop. The interaction between Asp30α of B7 and pTyr5 was found to be very strong, with a of −3.8 kcal mol −1 for a double-mutant cycle using alanine at position 5 ( Fig. 6a ). However, this cannot be attributable to the hydrogen bond to Asp30α, as a cycle with phenylalanine yielded a weak of only −0.2 kcal mol −1 . The interaction between Tyr104 of CDR3β and pTyr5 was stronger, with a of −0.8 kcal mol −1 . Although these cycles do not probe the entirety of B7 contacts to pTyr5, they are nonetheless instructive: engagement of pTyr5 by A6 is negligible, whereas it seems very favourable with B7. As the difference cannot be attributed to hydrogen bonds, it may arise from differences in packing and flexibility between the two TCRs, resulting in an entropic penalty with A6 not present with B7. This interpretation is supported by the specificities of the two TCRs: A6 tolerates a wide range of modifications to the centre of the peptide, yet B7 will only recognize targets with a tyrosine or a phenylalanine at position 5 (ref. 14 ). 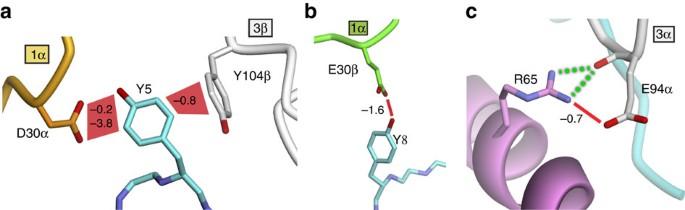Figure 6: Select interactions in the B7-Tax/HLA-A2 interface for comparison with similar interactions in the A6-Tax/HLA-A2 interface. (a) Engagement of pTyr5 of the Tax peptide is more substantive with B7 than with A6, but this is not attributable to hydrogen bonding. A double-mutant cycle between pTyr5 and Asp30 of CDR1α yielded an interaction free energy of −0.2 kcal mol−1with phenylalanine substituted for pTyr5. However, a cycle with alanine yielded a much more substantial value of −3.8 kcal mol−1. The interaction between pTyr5 and Tyr104 of CDR3β yielded a moderate interaction free energy of −0.8 kcal mol−1. (b) The hydrogen bond between Glu30 of CDR1β and pTyr8 of the Tax peptide is strong in the B7 interface, with an interaction free energy of −1.6 kcal mol−1. An identical interaction with the same strength is formed in the interface with A6 (Fig. 2b). (c) The hydrogen bond between Arg65 of the α1 helix and Glu94 of CDR3α in the interface with the B7 TCR is moderate, with an interaction free energy of −0.7 kcal mol−1. Arg65 also makes a bifurcated hydrogen bond with the carbonyl oxygen of Glu94, which as discussed in the text is also predicted to be stabilizing. Figure 6: Select interactions in the B7-Tax/HLA-A2 interface for comparison with similar interactions in the A6-Tax/HLA-A2 interface. ( a ) Engagement of pTyr5 of the Tax peptide is more substantive with B7 than with A6, but this is not attributable to hydrogen bonding. A double-mutant cycle between pTyr5 and Asp30 of CDR1α yielded an interaction free energy of −0.2 kcal mol −1 with phenylalanine substituted for pTyr5. However, a cycle with alanine yielded a much more substantial value of −3.8 kcal mol −1 . The interaction between pTyr5 and Tyr104 of CDR3β yielded a moderate interaction free energy of −0.8 kcal mol −1 . ( b ) The hydrogen bond between Glu30 of CDR1β and pTyr8 of the Tax peptide is strong in the B7 interface, with an interaction free energy of −1.6 kcal mol −1 . An identical interaction with the same strength is formed in the interface with A6 ( Fig. 2b ). ( c ) The hydrogen bond between Arg65 of the α1 helix and Glu94 of CDR3α in the interface with the B7 TCR is moderate, with an interaction free energy of −0.7 kcal mol −1 . Arg65 also makes a bifurcated hydrogen bond with the carbonyl oxygen of Glu94, which as discussed in the text is also predicted to be stabilizing. Full size image The B7 TCR utilizes the same Vβ 13-2 gene segment as A6, and the A6 and B7 CDR1β loops are positioned similarly over the peptide carboxy terminal end [31] . A double-mutant cycle between pTyr8 and Glu30β of B7 yielded a of −1.6 kcal mol −1 , identical within error to that measured between pTyr8 and Glu30β of A6 ( Fig. 6b ). Unlike the A6 TCR, the B7 CDR3β loop does not interact with pTyr8, which may explain the greater tolerance of B7 T cells to substitutions at position 8 (ref. 14 ). Nonetheless, the presence of a strongly favourable hydrogen bond from CDR1β to pTyr8 in both interfaces indicates that both TCRs arrive at the same germline loop-driven solution for optimizing electrostatic interactions with the peptide. Lastly, we examined engagement of Arg65 on the HLA-A2 α1 helix by B7. In the B7 complex, Arg65 forms a salt bridge with Glu94 of CDR3α, mimicking somewhat the salt bridge formed between Arg65 and Asp99 of the A6 CDR3α loop. However, compared with the highly favourable interaction formed in the A6 complex, the strength of the salt bridge with B7 was more modest, with a of only −0.7 kcal mol −1 . The differences between A6 and B7 likely reflect the suboptimal arrangement between the sidechains in the B7 interface ( Fig. 6c ). However, with B7, Arg65 also forms two hydrogen bonds with the carbonyl oxygen of Glu94α, which will likely provide additional favourable free energy. The existence of a favourable interaction between Arg65 and CDR3α of B7 is consistent with the observation that the B7 TCR does not recognize Arg65 mutants in functional assays [5] . Thus, both TCRs utilize CDR3α to productively engage Arg65 of the HLA–A2 α1 helix. Owing to their usual location in the centre of the interface, the central sidechains of a peptide are often assumed to be the focal point in antigen-specific TCR recognition. This is not the case with the A6 TCR: despite being accommodated in a central pocket with multiple hydrogen bonds, engagement of the sidechain of pTyr5 of the Tax peptide contributes little to binding. This observation helps explain a key aspect of A6 crossreactivity: the receptor tolerates significant alterations at the centre of the peptide [14] , [15] , with the CDR3β loop changing its conformation significantly with different peptides [13] , [15] , [16] , [18] , [19] . The high intrinsic flexibility of the A6 CDR3β loop [13] likely underlies the overall lack of stabilizing interactions between CDR3β and the peptide centre, as the entropic cost of ordering the loop will offset enthalpic gains from interatomic interactions. Crossreactivity in the A6 TCR can thus be attributed to a combination of flexibility and thermodynamic ambivalence (or entropy/enthalpy compensation) at the centre of the interface. This point is further established by the measurements with the B7 TCR: unlike A6, accommodation of pTyr5 by the B7 TCR is favourable. Yet the B7 TCR is less accommodating to substitutions at this position than A6 (ref. 14 ), and evidence suggests that the B7 hypervariable loops are less flexible than those of A6 (ref. 32 ). Although flexibility and thermodynamic ambivalence at the interface centre promotes A6 crossreactivity, this does not exclude a role for the peptide centre and its interactions with the TCR in defining some degree of specificity. A weak (or neutral) interaction is better than an unfavourable interaction, and the chemistry of the CDR3α/CDR3β loops and their accessible conformations will limit what sidechains will be tolerated. For example, A6 tolerates charged amino acids at position 5 of the peptide poorly [14] . Flexibility and thermodynamic ambivalence thus provides a mechanism for limited crossreactivity (or equivalently, limited specificity), a hallmark of T cell recognition. The TCR structural database indicates that TCR CDR loop flexibility is concentrated in the hypervariable loops [33] , indicating this strategy may be commonly utilized. In contrast with the peptide centre, pTyr8 near the C-terminal end dominates the peptide sidechain contributions to the binding of A6, demonstrating the impact peripheral peptide residues can have in TCR recognition. The interactions between the TCR and pTyr8 are a strong element of peptide specificity, as a tyrosine at position 8 is conserved in all known A6 agonists, and the interactions with the pTyr8 sidechain are among the few TCR–peptide interactions that are conserved in all ten crystal structures of A6 bound to a pMHC [10] , [12] , [13] , [14] , [15] , [16] , [18] , [19] . Comparing positions 5 and 8, the picture that emerges is that from a free-energy perspective, pTyr8 acts as a ‘lynchpin’ for binding of the A6 TCR, whereas pTyr5 is more of a neutral chemical ‘dollop’ around which the TCR moulds. It is notable that a significant amount of favourable energy resulting from engaging pTyr8 comes from the germline-encoded CDR1β loop, demonstrating the importance germline loops can have in determining antigen specificity. The observation that the B7 TCR utilizes CDR1β to make a similar stabilizing interaction with pTyr8 reinforces this point. Another striking observation is the dominance of the interactions between the A6 hypervariable CDR3α loop and the HLA-A2 α1 helix. This finding demonstrates conclusively that TCR hypervariable loops can have a significant influence on MHC restriction. Yet given the strength of these interactions, how is it that the A6 TCR maintains sufficient peptide specificity to have escaped the filtering process of negative selection? Crucially, the interactions between CDR3α and Arg65 cannot be considered in isolation, as their formation is dependent upon the peptide. In the bound state, the conformation the flexible A6 CDR3α loop adopts is dependent on the need to avoid steric clashes with other sidechains of HLA-A2 (ref. 13 ). However, this conformation can only be reached because of the glycine at peptide position 4: owing to steric crowding, any other amino acid would prevent CDR3α from adopting its bound conformation and making the crucial interactions with Arg65 ( Fig. 7 ). Indeed, A6 is intolerant of any amino acid other than glycine at position 4 (ref. 14 ). The peptide and MHC specificity of the A6 TCR are therefore inextricably linked. Although the extent to which similar results apply to other TCRs is unknown, this finding underscores the limitations of perspectives that consider MHC and peptide specificity as arising through independent mechanisms. 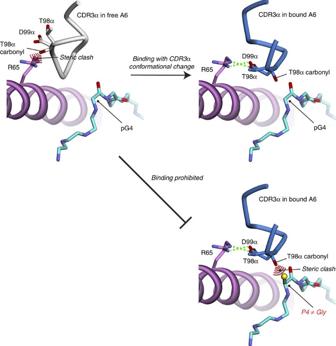Figure 7: The peptide and MHC specificity of the A6 TCR are inextricably linked. For TCR binding to proceed, the CDR3α loop must move from its position in the unbound structure to its position in the bound13. The conformational change is driven in part by a steric clash that would occur between the carbonyl oxygen of Thr98α and the sidechain of Arg65 (left panel). This conformational change permits formation of strongly stabilizing hydrogen bonds from Thr98α and Asp99α to Arg65 (top right). However, if an amino acid other than glycine were present at peptide position 4, a steric clash would occur between the Thr98α carboxyl and the position 4 β carbon (bottom right), preventing the loop from adopting its bound-state conformation and interacting with Arg65. Thus, formation of the strong interactions between CDR3α and Arg65 is dependent on the presence of glycine at peptide position 4. Glycine at position 4 is conserved in all known agonists for the A6 TCR. Figure 7: The peptide and MHC specificity of the A6 TCR are inextricably linked. For TCR binding to proceed, the CDR3α loop must move from its position in the unbound structure to its position in the bound [13] . The conformational change is driven in part by a steric clash that would occur between the carbonyl oxygen of Thr98α and the sidechain of Arg65 (left panel). This conformational change permits formation of strongly stabilizing hydrogen bonds from Thr98α and Asp99α to Arg65 (top right). However, if an amino acid other than glycine were present at peptide position 4, a steric clash would occur between the Thr98α carboxyl and the position 4 β carbon (bottom right), preventing the loop from adopting its bound-state conformation and interacting with Arg65. Thus, formation of the strong interactions between CDR3α and Arg65 is dependent on the presence of glycine at peptide position 4. Glycine at position 4 is conserved in all known agonists for the A6 TCR. Full size image The co-dependency of peptide and MHC specificity in the A6 TCR relates to the observation that the interactions between the germline-encoded loops and the MHC α1/α2 helices range from only moderately favourable to moderately unfavourable. This includes germline–MHC interactions that are shared in interfaces formed with multiple Vα 12-2 TCRs [29] , [30] . The extent to which evolution has influenced interactions between TCR germline loops and MHC proteins is controversial [34] , [35] . As discussed above though, weak interactions do not necessarily imply a lack of specificity. One interpretation consistent with our data is that rather than selecting for residues that will strongly stabilize the interaction of a TCR with an MHC, evolution has selected for sequences and conformations that can add some degree of stabilization when germline loops are docked alongside the MHC α helices, but can also ‘give’ when stronger interactions can be made elsewhere [35] , [36] . An evolutionarily selected permissiveness could explain not only the lack of strongly favourable germline–MHC contacts in the interfaces explored here, but also observations of non-canonical TCR-binding modes [37] , the finding that changes to a peptide alone can alter receptor-binding geometry [24] , the impact different CDR3 loops can have on TCR–MHC contacts [38] and the observation that TCRs that have not undergone selection can engage non-MHC targets [39] . It can also explain functional consequences of CDR2α mutations [40] , as these will perturb the energetic balance that leads to permissiveness. Such permissiveness may be a strategy for ensuring that any given TCR is able to best optimize its interactions with the composite peptide/MHC surface, and provided it is still able to engage with a conducive geometry [22] , initiate T cell signalling. Proteins and peptides TCRs and MHC proteins were refolded from bacterially expressed inclusion bodies according to established procedures [11] . TCRs utilized an engineered disulphide bond across the constant domains to ensure stability [41] . Amino acids targeted for mutations were identified from the TCR–pMHC structures using a 4 Å cutoff. Mutations were generated from the wild-type plasmids using PCR mutagenesis and confirmed by sequencing, or in some cases were available from previous studies [5] , [8] , [42] . Peptides were either synthesized in-house via solid-state synthesis using an ABI 433A instrument, or synthesized and purified commercially (Genscript). Double-mutant cycles In a double-mutant cycle, the interaction free energy between two amino-acid sidechains is determined via four measurements. The first measures the Δ G ° for the interaction between the two wild-type proteins. The second measures the effect of a single mutation on binding free energy ( ) and the third measures the effect of a second mutation ( ), typically at a position that interacts with the site of the first. The fourth measurement measures the effect of both mutations simultaneously ( ). The measurements refer to a cycle as shown in Fig. 1a . If there is no interaction (or coupling) between the two mutated sites, then the consequences of both mutations simultaneously is equal to the sum of the consequences of first and second mutations alone. Subject to the caveats described below, the extent to which this relationship does not hold defines the free energy of interaction between the two sidechains, that is: which simplifies to: where is the double-mutant binding free energy, the binding free energy for the first single mutant, the binding free energy for the second single mutant and the binding free energy for the wild-type proteins. Surface plasmon resonance data collection and analysis Double-mutant cycles were performed with surface plasmon resonance utilizing a Biacore 3000 instrument. Each cycle was performed with a strategy in which all four measurements (wild type, first single mutant, second single mutant and the double mutant) were performed in one experiment and fit globally. Wild-type and mutant TCR were coupled to adjacent flow cells. Coupling levels were between 400 and 1,200 RU. Two identical concentration series of wild-type and mutant pMHC were then simultaneously injected over both flow cells in succession, using concentrations as high as 400 μM, resulting in eight data sets for each cycle. All binding experiments were performed at 25 °C in 150 mM NaCl, 3 mM EDTA, 25 mM HEPES, 0.005% P-20, pH 7.4 using a steady-state equilibrium approach [11] . Data were processed with BiaEvaluation 4.1. For data analysis, after subtraction of the signal from a third blank flowcell, the eight data sets for each cycle were simultaneously fit to a model in which the four Δ G ° values and the surface activities of the two flow cells were fitted parameters. Global fitting as was performed with custom scripts in OriginPro 7.5 or 9.0. This strategy provides significant advantages over the traditional approach in which individual measurements are made and each cycle constructed from independent experiments, as it allows the determination of highly accurate ΔΔ G ° and values. Constraining the surface activities to values common to multiple data sets in which one has higher affinity than the other greatly increases the affinity range of surface plasmon resonance [43] , an advantage important for weak interactions involving mutants. Global fitting of multiple data sets reduces the influence of data set variation, enforces consistency and reduces parameter correlation [44] . Lastly, when the same sensor surfaces and dilution series are utilized in a titration, systematic errors such as instrumental noise and inaccuracies in protein concentration cancel when differences in free energies (that is, ΔΔ G ° and values) are computed. This last point is crucial, as noise and concentration errors contribute significantly to the error and uncertainty in low affinity measurements, as they have a disproportionate impact on regions of a binding curve that show large curvature. Note that because of this, in some cycles the measurements of ΔΔ G ° and may be more accurate than the individual Δ G ° measurements comprising it, a caveat that has no impact on our results. In almost all cases, the mutations in each double-mutant cycle were to alanine. As indicated in Supplementary Tables S1 and S2 , exceptions were leucine and valine for Q30α of A6 (as the Q30αA mutant expressed poorly), asparagine for D99α of A6 (to verify the strength of the interaction with R65 as described below), both alanine and phenylalanine for pY5 and pY8 (to investigate contacts to the tyrosine hydroxyl versus contacts to the aromatic ring) and glycine for A69 of HLA-A2. In addition, cycles involving K66 of HLA-A2 were performed in the background of the E63Q mutation to avoid complications arising from the complex electrostatic environment at this position [8] . In B7, both alanine and phenylalanine were substituted for pY5 to explore hydrogen bonding versus packing. Also with B7, we utilized asparagine for Asp30α, as the D30αA mutant expressed poorly. With the A6 TCR, five cycles yielded data in which the affinity of one or more interactions was too weak to yield an accurate value of (cycles in which Asp99α was mutated to alanine and three of four cycles in which pPhe8 was replaced with alanine or phenylalanine). These cycles were repeated with the high-affinity TCR variant A6 c134 (CDR3β: 99 MSAE 102 ) [20] or the fluorinated high-affinity Tax peptide variant Y5F FF [16] . The Y5F FF substitution has been shown previously to act independently of other substitutions in the interface, and select cycles performed with and without the A6 c134 variant yielded the same conclusions. Further, as shown in Supplementary Tables S1 and S2 and described in the main text, the conclusions from the A6 D99α—HLA-A2 R65 and A6 E30β—Tax pY8 cycles with the high-affinity variants were the same when performed in the wild-type background but instead substituting asparagine for D99 and alanine for pY8. The experiments with the DMF5 TCR utilized the high-affinity D26αY/L98βW variant [27] . In some instances (for example, Fig. 4b ), we consider the effects of double-mutant cycles in groups, a consideration that implicitly assumes additivity between the measurements. The extent to which additivity is permissible depends upon how well the chief assumptions in double-mutant cycles hold, that is, that the mutations are structurally independent and that any perturbations resulting from mutations are the same in the two single-mutant interfaces and the double-mutant interface [9] . While these necessarily limiting assumptions are unlikely to be valid in every instance, they have been supported when explicitly explored [45] . Support here can be found in the cases where very similar or even identical measurements were obtained when cycles were repeated using different amino acids at a single position (that is, Q30α-pL1, S31α-pY5, D99α-R65, E30β-pY8 and R95β-pY5 in the A6 interface). These measurements probed a range of environments, including those with complex electrostatics (D99α-R65) and high intrinsic flexibility (R95β-pY5). Error propagation of values was performed using standard statistical error propagation methods [11] . When multiple measurements were available, the values in the text and figures were the averages of the multiple measurements. How to cite this article: Piepenbrink, K. H. et al. The basis for limited specificity and MHC restriction in a T cell receptor interface. Nat. Commun. 4:1948 doi: 10.1038/ncomms2948 (2013).